Genetic architecture supports mosaic brain evolution and independent brain–body size regulation The mammalian brain consists of distinct parts that fulfil different functions. Finlay and Darlington have argued that evolution of the mammalian brain is constrained by developmental programs, suggesting that different brain parts are not free to respond individually to selection and evolve independent of other parts or overall brain size. However, comparisons among mammals with matched brain weights often reveal greater differences in brain part size, arguing against strong developmental constraints. Here we test these hypotheses using a quantitative genetic approach involving over 10,000 mice. We identify independent loci for size variation in seven key parts of the brain, and observe that brain parts show low or no phenotypic correlation, as is predicted by a mosaic scenario. We also demonstrate that variation in brain size is independently regulated from body size. The allometric relations seen at higher phylogenetic levels are thus unlikely to be the product of strong developmental constraints. The variation seen in overall brain size within and among species in relation to the size of different brain parts and of body size has been the focus of a large research effort because these fundamental relations reveal much about the constraints, adaptations and even candidate mechanisms that lead to micro- and macro-evolutionary change [1] , [2] , [3] , [4] . Several hypotheses based on comparative data have been developed to answer two fundamental questions about brain evolution [4] , [5] , [6] , [7] , [8] , [9] . The first is the degree to which the different functional brain systems evolve independently of each other and the brain as a whole. Under the mosaic evolutionary hypothesis, the size of different systems evolves independently due to differential selective pressures associated with different tasks [4] , [6] . In contrast, under a concerted evolutionary paradigm, promoted by Finlay and Darlington [1] , different regions are constrained or canalized by developmental factors and thus evolve predominantly as a whole. The distinction between these two hypotheses is central to our understanding of brain evolution and our interpretation of the underlying genetic, developmental and ecological mechanisms on which selection is presumed to operate. Comparative analyses of brain size have provided evidence for both hypotheses [1] , [6] , [10] . For example, the seminal data set collated and first analysed by Stephan et al . (for example, ref. 11 ) on brain and brain part sizes in primates and insectivores has provided the basis for much of the comparative analyses [2] . However, few studies, in particular in mammals, have investigated the genetic architecture of the brain to address the microevolutionary and genetic underpinnings of brain evolution [12] . Mosaic evolution of brain regions predicts that heritable variation in the size of different brain parts should be modulated by independent genetic loci and gene variants, and that phenotypic correlations among different brain parts may be low or absent. In contrast, under concerted evolution overlapping sets of loci should modulate the size of multiple parts of the brain with high levels of positive covariation. Quantitative genetic studies in the cave fish have demonstrated independent loci regulating the evolution of different eye phenotypes and argue in favour of a mosaic model [12] . A quantitative genetic approach offers the further advantage that the degree of mosaic versus concerted evolution may be inferred by comparing the level of variation explained by loci that are shared across many brain parts versus the level of variation explained by unique loci specific to brain parts. Although macroevolutionary patterns (for example, phylogenetic patterns seen above the species level including the occurrence of higher taxa) arise from microevolutionary mechanisms, that is, changes occurring within species [13] , it remains unclear whether specific brain parts can respond individually to selective pressure or are constrained in their response imposed by other brain parts or overall brain size. A second fundamental question is how phylogenetic differences in brain:body ratios have evolved. What are the mechanisms underlying the strong allometry between brain and body? Overall, brain size scales with body size due to linked processes very early during development [14] . After this initial phase, however, body size increases while brain size remains relatively constant [14] . Evolutionarily, the large relative brain to body size ratio, especially seen in many vertebrates, could in principle be due to changes in overall brain size or be secondary to changes in body size. It is evident that macroevolutionary trends among major vertebrate taxa have often involved a genuine increase in relative brain size at a constant body size, and that this has been made possible due to major changes in bioenergetics and life history [5] . However, at a microevolutionary level within species, brain size may be free to change independently of body size, with different genetic loci accounting for variation in the two traits and low phenotypic correlation between them. Here, we address these two key questions and present results of a 15-year research effort into the genetic architecture of brain and body size using a massive neuro-morphometric data set for ~10,000 mice belonging to a large set of recombinant inbred strains. The BXD family consists of ~100 lines derived from parental strains that differ at ~5 million single-nucleotide polymorphisms (SNPs), indels, transposons and copy-number variants [15] . This model system harbours naturally occurring genetic variation at a level approximating that of human populations. Our study utilizes a high-density linkage analysis [16] , [17] to map loci modulating phenotypic variation in overall brain size, body size and the size of seven major brain parts: the neocortex, cerebellum, striatum, olfactory bulb, hippocampus, lateral geniculate nucleus and basolateral complex of the amygdala. We scanned the entire genome, except the Y chromosome, using interval mapping as implemented in GeneNetwork ( http://www.genenetwork.org [17] ). Mapping relies on a set of 3,800 fully informative SNPs and microsatellite markers. In a second analysis, we scan the genome for all two-way epistatic interactions between loci. 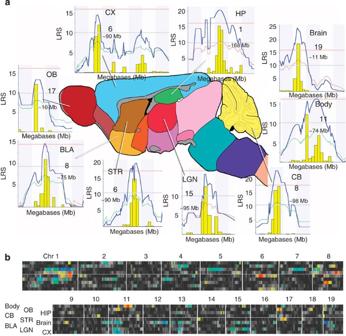Figure 1: Mouse brain sketch highlighting the analysed brain parts. (a) For each of the brain parts and body weight we show the corresponding genome scan with peaks identifying main loci, their location and chromosome number. Where individual peaks are shown, the red lines denote genome-wide significance and the grey line is the suggestive threshold. (b) The quantitative trait locus cluster maps provide a global whole-genome summary of mapping results for all key traits in the form of colour-coded horizontal bands—one per trait, extending from proximal chromosome 1 to distal chromosome X. Regions of more intense colour correspond to linkage peaks and the colours also encode whether the B allele (blue) or the D allele (red) contributes to large weight and volume. Body, body weight; BLA, basolateral complex; brain, overall brain weight; CB, cerebellum; CX, cortex; HP, hippocampus; LGN, lateral geniculate nucleus; OB, olfactory bulb; STR, striatum. Regulation of brain part size Our results show that distinct loci modulate the size of the brain, different brain regions and body size ( Table 1 , morphometric data are given in Table 2 ). Three loci on chromosomes 12, 15 and 19 influence variation in overall brain size ( Brain12a, Brain15a , Brain19a ; Fig. 1 ) and 15 loci modulate weights and volumes of specific brain regions. With one exception, no locus was shared among the seven brain parts nor with overall brain size. The sole exception involved a locus on mouse chromosome 6 that may jointly modulate the volume of both the striatum and neocortex ( Str6a and Cx6a ). We detected two epistatic interactions—one between Brw15a and Brw19a for overall brain weight and one between Str6a and Str17a for the striatum. With these two exceptions, we found no evidence for positive or negative gene-by-gene interaction between loci affecting overall brain size and those affecting the size of different brain parts. As no sets of loci were shared among brain parts or with overall brain size, we did not calculate the proportion of phenotypic variation accounted for by shared versus non-shared loci. Table 1 Loci for brain and body size traits. Full size table Table 2 Morphometric data. Full size table Figure 1: Mouse brain sketch highlighting the analysed brain parts. ( a ) For each of the brain parts and body weight we show the corresponding genome scan with peaks identifying main loci, their location and chromosome number. Where individual peaks are shown, the red lines denote genome-wide significance and the grey line is the suggestive threshold. ( b ) The quantitative trait locus cluster maps provide a global whole-genome summary of mapping results for all key traits in the form of colour-coded horizontal bands—one per trait, extending from proximal chromosome 1 to distal chromosome X. Regions of more intense colour correspond to linkage peaks and the colours also encode whether the B allele (blue) or the D allele (red) contributes to large weight and volume. Body, body weight; BLA, basolateral complex; brain, overall brain weight; CB, cerebellum; CX, cortex; HP, hippocampus; LGN, lateral geniculate nucleus; OB, olfactory bulb; STR, striatum. Full size image These results provide comparatively strong support for mosaic brain evolution. We can demonstrate that variation in the size of different brain parts is modulated by loci independent of each other and overall brain size. Although the different loci that control the size of brain parts may respond to selection in a similar manner, selection for specific tasks associated with individual brain parts renders micro-evolutionary change of the size of specific brain parts possible. We can further investigate the degree of independent regulation by analysing covariation between overall brain size and brain part size (both corrected for sex and age) and among the seven different brain phenotypes (corrected for overall brain size). Surprisingly, we found absent or low levels of correlation, ranging from −0.22 (Pearson's r ) between the olfactory bulb and basolateral geniculate nucleus to 0.29 between the olfactory bulb and cerebellum ( Table 3 ). Moreover, while the correlations between overall brain size and brain part size are always significant, they are intermediate and the associated r 2 values range from 0.12 to 0.55. For individual brain parts, these results suggest very little shared underlying genetic control. Indeed, the result of the quantitative genetic analysis showing independent regulation of overall brain size and brain part size, and among brain parts, is borne out by the phenotypic covariance analysis. Table 3 Partial correlation for relative size of brain parts. Full size table Brain and body size regulation We next addressed the second fundamental question of how the large relative brain size in mammals may have evolved by scanning the genome for loci that affect variation in body size to compare with those for overall brain size. We found evidence for independent loci governing brain and body size, the variation in which was affected by loci on different chromosomes, and no positive or negative epistatic interaction (indicative of potential constraints) was detected ( Table 1 ). Indeed, the phenotypic correlation between body size and overall brain size is very low, with only 3.3% of variation in brain size accounted for by variation in body size. These results suggest that variation in overall brain size is regulated by different underlying genes than is body size, with few genetic constraints on independent evolution of brain and body size. This conclusion is in agreement with results from comparative studies. Weston and Lister [8] could demonstrate that in dwarf hippopotami brain size reduction is much greater than body size reduction, which suggests that selective pressures on brain and body size can operate independently and cause deviations from traditional scaling models [8] . Further, a recent comprehensive systematic analysis in primates has shown that brain size decreased in a number of primate lineages [18] and found evidence for a dissociation between brain and body size at a macroevolutionary level. Our study demonstrates the necessary independent genetic regulation of brain and body size that may underlie the findings of these studies. In sum, our dissection of within-species variation provides compelling evidence for a mosaic control of brain region size as predicted by ecological and selection theory [19] . We do not suggest that the strong allometric patterns described by Finlay and Darlington cannot be explained by developmental/ontological processes and scaling functions at a macroevolutionary level. Indeed, Thompson [20] developed numerous functions that elegantly describe the relation between functionally very different structures. However, macroevolutionary patterns have microevolutionary origins [21] , [22] , [23] , [24] , [25] and at this level our results do not support strong developmental constraints. Specifically, we argue that apparent constraints seen at the macroevolutionary level do not mean that brain parts are necessarily constrained in their response to selection, nor that some parts may be spandrels (that is, a by-product of the evolution of other parts adapted later to specific tasks [2] , [26] ). This argument does not preclude the possibility that brain development may influence the direction of evolution on a larger scale by changing selectable phenotypic variation (refs 27 , 28 ) but it is clear that at a micro-evolutionary level brain part size can respond to selection in a largely independent way. The apparent constraints seen at higher phylogenetic levels are thus unlikely to be the product of strong developmental constraints and appear to mask discrete and mosaic selection. Subjects and phenotypes For our study we used over 10,000 individuals from the BXD panel of recombinant inbred lines. This family of mouse strains is segregating for ~5 million SNPs, indels and copy-number variations; a level of common sequence variation that matches or exceeds that in large human families and populations [17] . Over the past 15 years we have measured the overall brain weight, cerebellum, hippocampus, olfactory bulb weights and neocortex, basolateral complex, lateral geniculate nucleus and striatum volume and body weight from a total of 91 of these BXD lines [29] , [30] , [31] . In this work, we have adjusted brain phenotypes for age, sex, epoch and body weight. All histological data for this study were obtained from the Mouse Brain Library—a physical and internet resource that contains high-resolution images of histologically processed slides from over 3,200 adult mouse brains ( http://www.mbl.org ) with roughly balanced numbers of male and female specimens. The ages ranged from 21 to 694 days of age (mean±s.e.m.=103±5), with most of the cases ranging from 50 to120 days. Mice were obtained from either the Jackson Laboratory (Bar Harbor, ME, USA) or the University of Tennessee Health Science Center. All procedures were approved by the Institutional Animal Care and Use Committees and conform to the NIH guidelines for humane treatment of animals. Mice were deeply anesthetized with Avertin (0.8 ml intraperitoneal) and transcardially perfused with 0.9% saline, followed by fixative (1.25% glutaraldehyde/1.0% paraformaldehyde or 4% paraformaldeyde), and their brains removed and weighed. After variable post-fixation times, the brains were embedded in 12% celloidin and sliced in either a coronal or horizontal plane at a width of ~30 μm. Actual section thickness was determined by direct examination of 10 sections for each brain using an X100 oil immersion objective and a z axis micrometre. Estimation of regional volume The volume of brain regions was estimated using a computer controlled microscope (Nikon E800, Nikon, Inc., Melville, NY, USA) and Stereo Investigator (MBF Biosciences, Williston, VT, USA). Brain regions were parcellated by the criteria of the Allen Brain Atlas ( http://mouse.brain-map.org ). Volume was estimated by point counting using Cavalieri's method [32] . In cases where there were missing or damaged sections, a piece-wise parabolic estimation was used [33] . Final volume estimates were individually corrected for histological shrinkage by determining the previously computed ratio between the brain volume at fixation (brain weight) and that after processing. Genetic analysis The quantitative genetic analysis was performed using interval mapping and a set of 3,795 informative SNP markers across all chromosomes, except for the Y chromosome. We used the WebQTL mapping module in GeneNetwork ( http://www.genenetwork.org [17] , [34] ). Loci were identified by computation of likelihood ratio statistic scores, and significance was determined using 2,000 permutations of the phenotype data [35] . We further investigated two-locus epistatic interactions by searching for all possible interactions between pairs of loci in the genome. Phenotypes were then randomly permuted 500 times and reanalyzed using the pair-scan algorithm. We extracted the single highest likelihood ratio statistic (a measurement of the association between differences in phenotypes and differences in DNA sequence) for the full model for each of these permuted data sets. If the full model exceeded the permutation-based significance threshold, then different models for those locations can be tested by conventional χ 2 -tests at P <0.01. For both the interval mapping and epistasis analysis, we calculated thresholds at the suggestive ( P =0.63) and significant associations ( P =0.05 and P =0.01). How to cite this article: Hager, R. et al . Genetic architecture supports mosaic brain evolution and independent brain–body size regulation. Nat. Commun. 3:1079 doi: 10.1038/ncomms2086 (2012).